Cerebrospinal fluid-derived Semaphorin3B orients neuroepithelial cell divisions in the apicobasal axis The spatial orientation of cell divisions is fundamental for tissue architecture and homeostasis. Here we analysed neuroepithelial progenitors in the developing mouse spinal cord to determine whether extracellular signals orient the mitotic spindle. We report that Semaphorin3B (Sema3B) released from the floor plate and the nascent choroid plexus in the cerebrospinal fluid (CSF) controls progenitor division orientation. Delivery of exogenous Sema3B to neural progenitors after neural tube opening in living embryos promotes planar orientation of their division. Preventing progenitor access to cues present in the CSF by genetically engineered canal obstruction affects the proportion of planar and oblique divisions. Sema3B knockout phenocopies the loss of progenitor access to the CSF. Sema3B binds to the apical surface of mitotic progenitors and exerts its effect via Neuropilin receptors, GSK3 activation and subsequent inhibition of the microtubule stabilizer CRMP2. Thus, extrinsic control mediated by the Semaphorin signalling orients progenitor divisions in neurogenic zones. In multicellular organisms, the orientation of the cell division axis is essential for tissue architecture, function and homeostasis [1] . Up to now, the intrinsic molecular machinery positioning the mitotic spindle and its coupling to intrinsic cell polarities retained much attention [2] , [3] , [4] . Astral microtubules play a key role in division orientation by linking the mitotic spindle to the cell cortex and transmitting pulling forces to trigger the spindle motion. The position of astral microtubule anchorages at the cell cortex largely depends on intrinsic localized cortical proteins such as the leucine-glycine-asparagine repeat protein LGN or cell polarity proteins that recruit dynein/dynactin motor complex. However, several lines of evidence suggest that the setting of the cell division axis also receives external influence [5] , [6] . The planar polarity pathway transmits to individual progenitors the general polarity of the tissue through cell-to-cell interactions. This polarity serves as a landmark for the orientation of divisions [7] . Apart from the planar polarity pathway, very little is known on other contributions of extracellular cues, their sources and identity, the nature of the information they provide to dividing cells and their links with the intrinsic cell machinery. In the developing vertebrate neural tube, early neural progenitors are organized into a neuroepithelium closed around a central canal. The dorsal and the ventral organizing centres of the neural tube, the roof plate and the floor plate, respectively, are major sources of extracellular cues [8] . By releasing morphogens in the central canal they play a crucial role in the specification of progenitor and post-mitotic cell lineages. Interestingly, the neuroepithelial cells align along the apicobasal axis and their nuclei migrate between the apical and the basal poles through the cell cycle. Mitosis occurs when the nucleus is at the apical pole, close to the canal, and at the S phase when the nucleus is at the basal pole [9] . Thus, signals from the canal could be delivered to mitotic progenitors to orient their division axis. In the developing vertebrate neuroepithelium, a complex mosaic of progenitor populations divides asynchronously to generate neural cells with distinct fates [10] . The orientation of neural progenitor division is generally categorized as planar, when the division plane is parallel to the apicobasal axis or oblique in other cases [10] , [11] . However, this binary classification may mask a diversity of mitotic spindle orientation proceedings reflecting the concomitance of various neural progenitor populations. Depending on the progenitor types, the divisions give rise to either two neurons, or one progenitor and one neuron, or to two progenitors, the daughter progenitors reproducing or not mother cell division mode [11] , [12] . Although this great diversity of dividing cells is not yet distinguishable by molecular markers, specific controls might exist for each of these co-existing progenitor divisions, which have not been investigated yet. In the present study, we report that the distribution of division angles in the neuroepithelial tissue at the onset of neurogenesis is highly stereotyped, suggesting that it might be tightly controlled at the tissue level. We investigated whether such control could arise from extracellular cues. Through combinations of in vivo and ex vivo approaches we show that Semaphorin3B (Sema3B), a cell and axon guidance molecule [13] , [14] , is released in the cerebrospinal fluid (CSF) by a ventral tissue lying in the central canal, the floor plate and the forming choroid plexus, and is delivered to apical progenitors undergoing mitosis. This signal is required for setting the stereotyped distribution of division angles. These data reveal first that CSF-derived extrinsic factors control the apicobasal orientation of cell divisions and second bring to light a novel and unexpected contribution of the Semaphorin signalling during the early steps of neural development. Apicobasal orientation of progenitor division is stereotyped We assessed how the division orientation of neural progenitors with respect to the apical plane is distributed within the spinal neuroepithelium during neurogenesis. Pioneer studies in the field assessed the orientation division on two-dimensional images of tissue sections, which could strongly distort the value of the division plane leading to overestimation of the percentage of oblique divisions. To obtain a precise determination of the division orientation, the angle between the cell division and apical planes was calculated from high-resolution three-dimensional (3D) confocal stacks of dividing cells (see Methods). At E10.5, remarkably, the proportion of the division angles of spinal neuroepithelial cells was very similar between embryos from different genetic backgrounds such as C57Bl6/J and OF1 ( Supplementary Fig. 1 ). This indicated that our angle analysis protocol was sensitive and robust. Although most (65%) divisions showed planar (80°–90° class) orientation, we also observed a diversity of oblique angle classes, mostly restricted between 50° and 80°, suggesting a control of division orientations specific of progenitor subsets. Previous studies often classified their angle in three classes (0–30°, 30–60° and 60–90°). However, we observed that angles between 80° and 90° are largely predominant to angles ranging between 60 and 80° ( Supplementary Fig. 1c ), indicating that two distinct cell classes may exist and be differently regulated for their division orientation. This prompted us to define 80–90° and 60–80° angle classes in the following analyses. Sema3B is secreted in the central canal of the spinal cord Mitotic spindle orientation largely relies on astral microtubules and cortical actin cytoskeleton [15] , [16] . We hypothesized that extracellular signals known to regulate actin and microtubule dynamics, such as axon guidance cues, could be good candidates to influence cell division orientation. Interestingly, axon guidance cues play very specific effects, acting on restricted cell subpopulations. Distinct neuronal pools display variable sensitivity to such cues, which thus allows them to adopt specific behaviours. Semaphorin family members, among which the secreted Sema3B , are expressed at the ventral border of the canal, by the time axons navigate in the spinal cord at E11.5 (refs 13 , 14 , 17 , 18 ). Interestingly, we could detect earlier Sema3B mRNA expression, at E9.5 and E10.5 in the floor plate and in the notochord ( Fig. 1a ). Remarkably in the brain, the choroid plexi, which secrete signals in the CSF, were other prominent sources of Sema3B. From E10.5 Sema3B , mRNA was detected in the nascent choroid plexus of the IVth ventricle, and this expression spanned later on to all choroid plexi of the brain ( Fig. 1a and Supplementary Fig. 2 ). To characterize the Sema3B protein distribution, we engineered a Sema3B-GFP (green fluorescent protein) knock-in mouse line in which the enhanced GFP (EGFP) was fused to the N-terminal end of Sema3B ( Supplementary Fig. 3 ). Anti-GFP immunostaining on E10.5 cryosections revealed signal lining the ventricle in floor plate cells and in the notochord ( Fig. 1b ). Interestingly, Sema3B protein accumulated at the apical pole of floor plate cells, suggesting that it is sorted for secretion in the central canal. Comparable knock-in gfp mouse model led to the observation that the floor plate cue Sonic hedgehog diffused laterally in the spinal cord walls, establishing a dorsoventral gradient [19] . Such lateral diffusion of Sema3B was not observed in Sema3B-GFP sections, as indicated by plot profile analysis of the GFP signal ( Fig. 1b ). When isolated floor plates from Sema3B-GFP KI embryos were cultured for 2 days, Sema3B-GFP could be detected in the conditioned medium ( Fig. 1c ). Moreover, endogenous Sema3B-GFP protein could be detected by western blotting of samples of CSF harvested in the IVth ventricle of E10.5 Sema3B-GFP KI embryos ( Fig. 1d , Supplementary Fig. 3 ). Thus, Sema3B can be released from the floor plate and the nascent choroid plexi in the central canal. 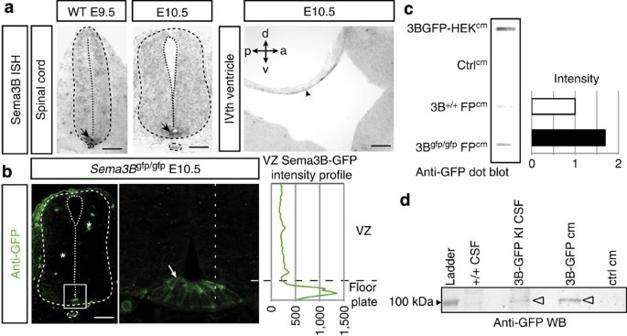Figure 1: Sema3B is expressed in floor plate cells of the spinal cord at stages E9.5–E10.5 and in the presumptive choroid plexus of the IVth ventricle at E10.5. (a)In situhybridization ofSema3BmRNA on mouse spinal cord cross-sections at E9.5–E10.5 and sagittal section at the hindbrain roof level at E10.5 (arrow, floor plate; arrowhead, roof of the IVth ventricle presumptive of the choroid plexus; a, anterior; p, posterior; d, dorsal; v, ventral). (b) Confocal images of GFP immunostaining on Sema3Bgfp/gfpspinal cord sections at E10.5. Intensity plot profile of Sema3B-GFP staining along the ventricular zone and the floor plate (dotted line). Strong Sema3B-GFP staining is detected in the spinal floor plate. Note the strong accumulation at the apical side of floor plate cells (arrow). No Sema3B-GFP gradient was detected along the dorsoventral axis within the ventricular zone (VZ). Stars indicate unspecific fluorescence in blood vessels. Scale bars ina,b, 100 μm. (c) Anti-GFP slot blotting of conditioned medium from Sema3B-GFP-transfected HEK293T (3BGFP-HEKcm) cells and WT (3B+/+FPcm) andSema3Bgfp/gfpfloor plates (3Bgfp/gfpFPcm). Chemiluminescence intensities of this representative case were quantified (histograms at right). Sema3B-GFP is detected in FPcmfromSema3Bgfp/gfpembryos. Similar results were obtained in two independent experiments. (d) Anti-GFP western blotting on the cerebrospinal fluid from E10.5Sema3B-GFPKI embryos collected at the level of the IVth ventricle. In theSema3B-GFPKI CSF, we observed a specific band (white arrowheads) of ~110 kDa corresponding to the full-length Sema3B fused to GFP. CSF from E10.5 wt OF1 embryos is used as a negative control, conditioned medium from Sema3B-GFP-transfected HEK cells as a positive control of anti-GFP antibody specificity. Figure 1: Sema3B is expressed in floor plate cells of the spinal cord at stages E9.5–E10.5 and in the presumptive choroid plexus of the IVth ventricle at E10.5. ( a ) In situ hybridization of Sema3B mRNA on mouse spinal cord cross-sections at E9.5–E10.5 and sagittal section at the hindbrain roof level at E10.5 (arrow, floor plate; arrowhead, roof of the IVth ventricle presumptive of the choroid plexus; a, anterior; p, posterior; d, dorsal; v, ventral). ( b ) Confocal images of GFP immunostaining on Sema3B gfp/gfp spinal cord sections at E10.5. Intensity plot profile of Sema3B-GFP staining along the ventricular zone and the floor plate (dotted line). Strong Sema3B-GFP staining is detected in the spinal floor plate. Note the strong accumulation at the apical side of floor plate cells (arrow). No Sema3B-GFP gradient was detected along the dorsoventral axis within the ventricular zone (VZ). Stars indicate unspecific fluorescence in blood vessels. Scale bars in a,b , 100 μm. ( c ) Anti-GFP slot blotting of conditioned medium from Sema3B-GFP-transfected HEK293T (3BGFP-HEK cm ) cells and WT (3B +/+ FP cm ) and Sema3B gfp/gfp floor plates (3B gfp/gfp FP cm ). Chemiluminescence intensities of this representative case were quantified (histograms at right). Sema3B-GFP is detected in FP cm from Sema3B gfp/gfp embryos. Similar results were obtained in two independent experiments. ( d ) Anti-GFP western blotting on the cerebrospinal fluid from E10.5 Sema3B-GFP KI embryos collected at the level of the IVth ventricle. In the Sema3B-GFP KI CSF, we observed a specific band (white arrowheads) of ~110 kDa corresponding to the full-length Sema3B fused to GFP. CSF from E10.5 wt OF1 embryos is used as a negative control, conditioned medium from Sema3B-GFP-transfected HEK cells as a positive control of anti-GFP antibody specificity. Full size image Sema3B binds the apical pole of mitotic progenitors Since Sema3B is delivered to the CSF, we investigated whether the spinal progenitors possess Sema3B-binding sites. We opened E10.5 spinal cords and exposed their apical face to Sema3B-GFP or GFP control protein. We observed in 75% of the apical feet of progenitors numerous Sema3B-binding sites at their surface, accumulating in large central domains of the end feet but not at intercellular junctions ( Fig. 2b,c ). As a control, GFP staining was not observed deeper in the cell, confirming that it is restricted to the apical surface. 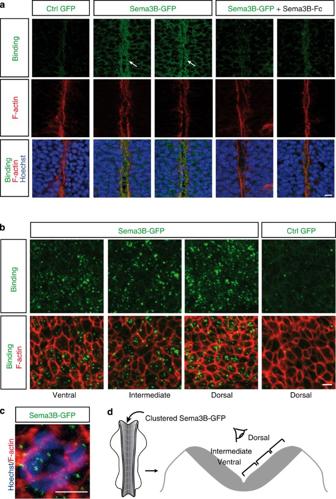Figure 2: Sema3B binds the apical surface of neuroepithelial cells of E10.5 spinal cords. (a) Confocal images of anti-GFP immunostaining showing binding sites of clusters of exogenous Ctrl GFP and Sema3B-GFP alone in transverse E10.5 sections, with competitive unlabelled Sema3B-Fc. Hoechst and phalloidin staining label, respectively, nuclei and neuroepithelium apical side. Specific Sema3B-GFP-binding sites strongly accumulated at the apical side (arrow) of neural progenitors. In addition, Sema3B-GFP-binding sites were also observed within the VZ. (b) Confocal images showing binding sites of clusters of exogenous Sema3B-GFP and Ctrl GFP in open-book configuration as depicted ind. Apical end feet of neural progenitors in the ventral, intermediate and dorsal parts of the spinal cord in planar view are delineated by phalloidin staining. (c) Higher magnification of a Sema3B-GFP-bound apical foot of an anaphase cell (underlying chromosomes were overlaid in blue). Scale bars (a), (b) 10 μm, (c), 5 μm. Figure 2: Sema3B binds the apical surface of neuroepithelial cells of E10.5 spinal cords. ( a ) Confocal images of anti-GFP immunostaining showing binding sites of clusters of exogenous Ctrl GFP and Sema3B-GFP alone in transverse E10.5 sections, with competitive unlabelled Sema3B-Fc. Hoechst and phalloidin staining label, respectively, nuclei and neuroepithelium apical side. Specific Sema3B-GFP-binding sites strongly accumulated at the apical side (arrow) of neural progenitors. In addition, Sema3B-GFP-binding sites were also observed within the VZ. ( b ) Confocal images showing binding sites of clusters of exogenous Sema3B-GFP and Ctrl GFP in open-book configuration as depicted in d . Apical end feet of neural progenitors in the ventral, intermediate and dorsal parts of the spinal cord in planar view are delineated by phalloidin staining. ( c ) Higher magnification of a Sema3B-GFP-bound apical foot of an anaphase cell (underlying chromosomes were overlaid in blue). Scale bars ( a ), ( b ) 10 μm, ( c ), 5 μm. Full size image Consistent with our findings on open books, Sema3B-GFP but not control GFP binding to the apical surface of the neuroepithelium was detected on unfixed coronal cryosections ( Fig. 2a ). Moreover, in the Sema3B condition, the GFP signal was strongly reduced by competition of Sema3B-GFP by Sema3B-Fc, thus confirming the Sema3B binding specificity ( Fig. 2a ). Thus, Sema3B has the secretion and binding profiles required to exert direct effects on neuroepithelial cells. Sema3B orients cell divisions in the apicobasal axis We thus addressed whether Sema3B could regulate the orientation of progenitor divisions. We designed an in vivo experimental paradigm. It consisted of a dorsal incision of living mouse embryos to open the central canal of the neural tube and to interfere with the delivery of CSF-derived extracellular cues. We reasoned that this manipulation should alter the distribution of the division angles, and if Sema3B has an instructive role in mitotic spindle orientation, then apical Sema3B exposure should restore the normal distribution of division angles. E10.5 embryos were opened or left intact for control, and recombinant Sema3B-Fc was applied on top of the open neural tube. Precautions were taken to avoid tissue-stretching. The embryos were maintained ex utero for 3 h in DMEM-F12/neurobasal medium ( Fig. 3a ). This timing allowed newly apical mitotic progenitors to be exposed to Sema3B-Fc in this spatial configuration from the prophase to the anaphase. Staining of the tight junction protein ZO1, and F-actin on open-book spinal cord maintained for 3 h in these culture conditions, confirmed that the apical feet and the pseudostratified organization of neural progenitors were preserved. In addition, labelling of the apical polarity proteins aPKC showed that the apicobasal polarity of neuroepithelial cells was not affected in the open-book neural tube ( Fig. 3e ). Caspase 3 immunostaining was also performed and it confirmed the absence of any abnormal death in open neural tubes after 3-h culture (data not shown). We then analysed the orientation of the mitotic spindle in anaphase neuroepithelial cells on cryosections. The percentage of planar divisions (90°–80°) was 42% decreased in open embryos compared with intact ones, with oblique divisions increasing to 67% of the total ( Fig. 3b–d and Supplementary Fig. 4 ). Cells with the horizontal division plane (0°–30°) were observed only under the open condition, and never in intact controls ( Fig. 3c ). Remarkably, Sema3B exposure could restore the distribution of division orientations observed in the intact embryos, by suppressing supernumerary-deviated divisions ( Fig. 3b–d ). These results reveal that the orientation of neuroepithelial cell division with respect to the apicobasal axis can be influenced by extracellular signals exposed to their apical pole. In addition, Sema3B is a potent extracellular factor promoting planar division orientation. 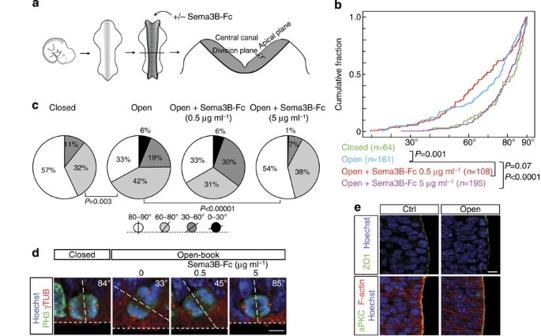Figure 3: Short-term exposure of spinal neural progenitors in the open-book configuration with Sema3B promotes the planar orientation of their division at E10.5. (a) Schema of the open-book surgery, Sema3B-Fc exposure and analysis of cell division orientation of spinal neuroepithelial cells in the apicobasal axis on transverse sections at the brachial and thoracic levels. (b) Cumulative fraction curves showing the distribution of apical progenitor division orientation in closed and open neural tubes exposed or not with recombinant Sema3B-Fc for 3 h at E10.5. (n, number of cells examined from at least three independent experiments and five embryos for each conditions,Pvalue is from the Kolmogorov-Smirnov (KS) test). (c) The same data sets are reported in pie charts with four classes displaying planar (80–90°) and oblique (60–80°, 30–60° and 0–30°) divisions of spinal progenitors (Pvalue is from Fisher’s exact test). (d) Confocal images of representative anaphase cells, with Hoechst, PH3 and γ-tubulin stainings. Division and apical planes are indicated in dotted lines (scale bar, 5 μm). (e) Staining of ZO1, F-actin, atypical PKC and Hoechst on cryosections of control embryos fixed without incubation or open-book embryos after 3-h culture. The apical architecture of the neuroepithelium in the open-book condition was preserved (scale bar, 10 μm). Figure 3: Short-term exposure of spinal neural progenitors in the open-book configuration with Sema3B promotes the planar orientation of their division at E10.5. ( a ) Schema of the open-book surgery, Sema3B-Fc exposure and analysis of cell division orientation of spinal neuroepithelial cells in the apicobasal axis on transverse sections at the brachial and thoracic levels. ( b ) Cumulative fraction curves showing the distribution of apical progenitor division orientation in closed and open neural tubes exposed or not with recombinant Sema3B-Fc for 3 h at E10.5. ( n , number of cells examined from at least three independent experiments and five embryos for each conditions, P value is from the Kolmogorov-Smirnov (KS) test). ( c ) The same data sets are reported in pie charts with four classes displaying planar (80–90°) and oblique (60–80°, 30–60° and 0–30°) divisions of spinal progenitors ( P value is from Fisher’s exact test). ( d ) Confocal images of representative anaphase cells, with Hoechst, PH3 and γ-tubulin stainings. Division and apical planes are indicated in dotted lines (scale bar, 5 μm). ( e ) Staining of ZO1, F-actin, atypical PKC and Hoechst on cryosections of control embryos fixed without incubation or open-book embryos after 3-h culture. The apical architecture of the neuroepithelium in the open-book condition was preserved (scale bar, 10 μm). Full size image Our previous data supported that Sema3B released ventrally from the floor plate in the central canal is delivered to progenitors lying at the central canal border during their mitosis. If this is true, then interfering with the canal fluid diffusion should have an impact on the progenitor division orientation. To assess this idea, we used a PGK:CRE;Dbx1-IRES-loxP-Stop-loxP-DTA mouse line [20] to ablate Dbx1+ progenitors lying in the spinal ventricular zone at the intermediate dorsoventral level. We observed that their genetic ablation resulted in ventricular border fusion at the site these progenitors normally occupy, starting at E10.5. This closure led to the formation of a double (ventral and dorsal) canal, which could impair the diffusion of secreted molecules between the ventral and dorsal compartments (we refer to this line as ‘double-canal line (DC)’, Fig. 4a and Supplementary Fig. 5 ). Nearby progenitors that did not express Dbx1 were unaffected in the DC line, showing normal expression of Olig2, Nkx2.2 and Pax7 (ref. 21 ; Supplementary Fig. 5 ). Sema3B expression in the ventral compartment was also preserved ( Supplementary Fig. 5 ). We analysed cell division orientation of progenitors residing in the dorsal and ventral compartments of E10.5 DC embryos, avoiding the cells in close vicinity with the fusion domain. In the DC mutants, the proportion of planar divisions was unchanged in the ventral compartment, indicating that Dbx1+ cell ablation and border fusion had no effect per se on progenitor division orientation ( Fig. 4b,c and Supplementary Fig. 4 ). In contrast, the proportion of planar divisions in the dorsal compartment of DC mutants was 77% of the normal dorsal compartment ( Fig. 4b,c ). Thus, as expected from our previous findings and Sema3B ventral origin, interfering with the canal flow affected the orientation of dorsal progenitor divisions. 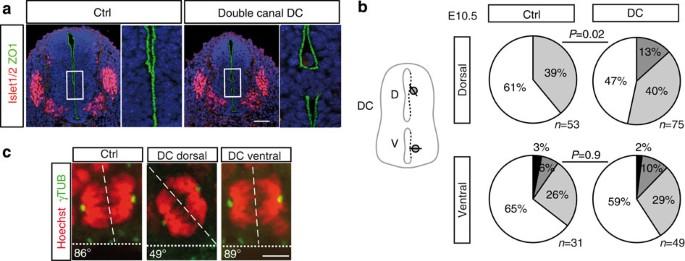Figure 4: Genetically interfering with dorsoventral diffusion of CSF-derived cues alters dorsal progenitor division orientation at E10.5. (a) ZO1 and Islet1/2 immunostaining on E11 WT and DC (PGK:CRE;Dbx1-IRES-loxP-Stop-loxP-DTA) spinal cord sections. (b) Proportions of planar and oblique divisions of ventral and dorsal progenitors in E10.5 WT and DC spinal cords as depicted in the schema (Pvalue is from Fisher’s exact test). (c) Confocal images of representative anaphase cells, with Hoechst and γ-tubulin immunostaining. Division and apical planes are indicated in dotted lines. Scale bars ina, 100 μm and inc, 5 μm. Figure 4: Genetically interfering with dorsoventral diffusion of CSF-derived cues alters dorsal progenitor division orientation at E10.5. ( a ) ZO1 and Islet1/2 immunostaining on E11 WT and DC (PGK:CRE;Dbx1-IRES-loxP-Stop-loxP-DTA) spinal cord sections. ( b ) Proportions of planar and oblique divisions of ventral and dorsal progenitors in E10.5 WT and DC spinal cords as depicted in the schema ( P value is from Fisher’s exact test). ( c ) Confocal images of representative anaphase cells, with Hoechst and γ-tubulin immunostaining. Division and apical planes are indicated in dotted lines. Scale bars in a , 100 μm and in c , 5 μm. Full size image Sema3B loss affects the stereotypical division orientation We then examined the in vivo consequences of the genetic knockout of Sema3B on the stereotypic profile of division orientations [14] . The percentage of planar divisions was reduced in favour of oblique divisions in E10.5 Sema3B −/− embryos compared with wild types. This effect was observed in the ventral but also in the dorsal ventricular zone ( Fig. 5a–c and Supplementary Fig. 4 ). Interestingly, we found similar division angle proportions between opened wild type and closed Sema3B −/− spinal cords after 3-h culture ( Supplementary Fig. 6 ). Thus, the response to Sema3B knockout mimicked the response to surgical opening of the neural tube, both procedures resulting in excessive oblique mitoses. Moreover, in contrast to wt, opening spinal cords of Sema3B −/− mutants did not further decrease the percentage of planar divisions ( Supplementary Fig. 6 ). This indicates that the loss of planar division consecutive to neural tube opening was mainly because of Sema3B depletion, consistent with a major role of Sema3B in promoting planar divisions at E10.5. Meanwhile, the contribution of other factors is possible, since opening the neural tube also decreased the 60°–80° class in favour of the more oblique 30°–60° one in the Sema3B −/− context ( Supplementary Fig. 6 ). 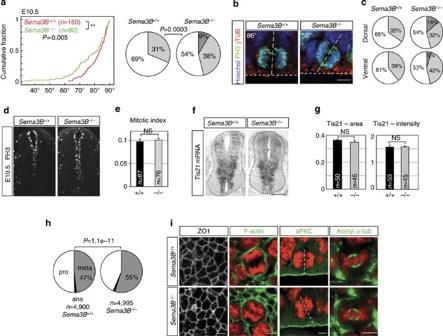Figure 5: Sema3B invalidation alters the orientation of neural progenitor divisions at E10.5. (a) Cumulative fraction curves showing the distribution of neural progenitor division orientation in E10.5Sema3B+/+and−/−spinal cords (n, number of cells from a minimum of five embryos per condition,Sema3B+/+and−/−embryos from the same litters were analysed;Pvalue is from the KS test). Previous data sets are also displayed in pie charts (Pvalue is from Fisher’s exact test). (b) Confocal images of representative anaphase cells with hoechst, PH3 and γ-tubulin stainings. (c) Planar and oblique division proportions in the ventral and dorsal halves of Sema3B+/+and Sema3B−/−spinal cords. (d) PH3 immunolabelling revealing mitotic cells in E10.5 Sema3B+/+and−/−spinal cord sections. (e) Mitotic index in E10.5Sema3B+/+and−/−spinal cord sections at the thoracic and brachial levels (n,number of sections from 10 embryos; ns not significant with Mann–WhitneyU-test). The number of mitotic progenitors is not altered by Sema3B invalidation at E10.5. (f)In situhybridization ofTis21mRNA in E10.5 Sema3B+/+and−/−spinal cord sections. (g)Tis21mRNA staining area and intensity at the thoracic and brachial levels (n,number of cross-sections from four embryos in each condition;Pvalue is from Mann–WhitneyU-test). (h) Proportions of prophases (Pro), metaphases (Meta) and anaphases (Ana) among mitotic progenitors of E10.5Sema3B+/+and−/−spinal cords at the thoracic and brachial levels. The percentage of metaphase cells is increased in E10.5Sema3Bmutants (n, number of PH3+ cells analysed from five embryos for each conditions.Sema3B+/+and−/−embryos were from the same litters). (i) Confocal images revealing ZO1 (planar view), aPKC (cross-section) stainings at the level of neural progenitors apical feet and F-actin and acetylated tubulin stainings in anaphase and metaphase neural progenitors (planar view) inSema3B+/+and−/−E10.5 spinal cords. Apical foot morphology, cortical actin and mitotic spindles are detected with similar patterns under both conditions. Scale bars inb,i, 5 μm, ind,f, 100 μm. Figure 5: Sema3B invalidation alters the orientation of neural progenitor divisions at E10.5. ( a ) Cumulative fraction curves showing the distribution of neural progenitor division orientation in E10.5 Sema3B +/+ and −/− spinal cords ( n , number of cells from a minimum of five embryos per condition, Sema3B +/+ and −/− embryos from the same litters were analysed; P value is from the KS test). Previous data sets are also displayed in pie charts ( P value is from Fisher’s exact test). ( b ) Confocal images of representative anaphase cells with hoechst, PH3 and γ-tubulin stainings. ( c ) Planar and oblique division proportions in the ventral and dorsal halves of Sema3B +/+ and Sema3B −/− spinal cords. ( d ) PH3 immunolabelling revealing mitotic cells in E10.5 Sema3B +/+ and −/− spinal cord sections. ( e ) Mitotic index in E10.5 Sema3B +/+ and −/− spinal cord sections at the thoracic and brachial levels ( n, number of sections from 10 embryos; ns not significant with Mann–Whitney U -test). The number of mitotic progenitors is not altered by Sema3B invalidation at E10.5. ( f ) In situ hybridization of Tis21 mRNA in E10.5 Sema3B +/+ and −/− spinal cord sections. ( g ) Tis21 mRNA staining area and intensity at the thoracic and brachial levels ( n, number of cross-sections from four embryos in each condition; P value is from Mann–Whitney U -test). ( h ) Proportions of prophases (Pro), metaphases (Meta) and anaphases (Ana) among mitotic progenitors of E10.5 Sema3B +/+ and −/− spinal cords at the thoracic and brachial levels. The percentage of metaphase cells is increased in E10.5 Sema3B mutants ( n , number of PH3+ cells analysed from five embryos for each conditions. Sema3B +/+ and −/− embryos were from the same litters). ( i ) Confocal images revealing ZO1 (planar view), aPKC (cross-section) stainings at the level of neural progenitors apical feet and F-actin and acetylated tubulin stainings in anaphase and metaphase neural progenitors (planar view) in Sema3B +/+ and −/− E10.5 spinal cords. Apical foot morphology, cortical actin and mitotic spindles are detected with similar patterns under both conditions. Scale bars in b , i , 5 μm, in d , f , 100 μm. Full size image Our findings that short-term Sema3B application could regulate the distribution of division angles suggested that the effect might be direct, rather than resulting from indirect alteration of the number of progenitors undergoing planar and oblique divisions. Would the effect be indirect, it could be due to earlier depletion of mitotic progenitors that normally would have undergone planar division or to increase in neurogenic progenitors dividing asymmetrically. Phospho-histone H3 (PH3) immunolabelling revealed that the number of M phase progenitors was normal in E10.5 Sema3B null embryos (Fig. 5d,e ). Tis21, a marker of neurogenic progenitors [22] , had comparable expression profile in E10.5 Sema3B −/− and +/+ embryos. Thus, the ratio of neurogenic/proliferative divisions was not affected by Sema3B loss ( Fig. 3f,g ). F-actin and acetylated tubulin staining did not reveal gross alterations of the cortical actin cytoskeleton and mitotic spindle, respectively, in Sema3B −/− mutants. We observed no abnormalities in the ventricular zone morphology, progenitor patterning. Progenitor adherens junctions, apical foot size and apical marker distribution were preserved in Sema3B −/− mutants, suggesting that the apicobasal polarity is not disrupted by Sema3B loss ( Fig. 5i and Supplementary Fig. 7 ). Thus, the loss of planar divisions might result from direct deregulation of the orientation of progenitor division. The final position of the mitotic spindle prefiguring the orientation of the cytokinesis is set at the metaphase [1] . A significant increase of 8% of cells in the metaphase among PH3+ progenitors could be detected in E10.5 Sema3B −/− embryos compared with their wild-type counterparts ( Fig. 3h ), which is consistent with a delay in metaphase and an alteration of the setting of division angles. Random division orientation in the spinal dorsoventral axis In the vertebrate nervous system, apicobasal orientation of progenitor division is tightly controlled [23] . We wondered whether some mechanisms exist that orient cell divisions along the dorsoventral axis and, if so, whether they require Sema3B, which is secreted ventrally. We analysed the cell division orientation at E10.5 and E11.5 in the dorsoventral dimension. In contrast to our observations in the apicobasal axis, classes of division angles are equally represented in the dorsoventral plane. Moreover, the distribution of progenitor division orientation in the DV-AP axes is not affected by Sema3B loss, neither in the ventral nor in the dorsal domains of the spinal cord ( Supplementary Fig. 8 ). Thus, topographic landmarks signalled by Sema3B are specific to the apicobasal axis. Sema3B genetic loss alters the timing of motoneuron birth In the cerebral cortex and the spinal cord, randomization of the orientation of neural progenitor division or bias towards very oblique angles is accompanied by ectopic localization of progenitors, proliferation and neurogenesis defaults [1] , [16] , [24] , [25] . We tested whether the effects of Sema3B loss on the division orientation were as drastic as those induced by manipulations of the intracellular effectors that position the spindles. We found that Sema3B loss did not lead to ectopic PH3+ cells in the mantle zone ( Supplementary Fig. 9 ). Thus, altering extracellular components that provides positional information to the progenitors is not detrimental to their apical anchorage. We then explored whether Sema3B loss has an impact on progenitor proliferation and neurogenesis in the spinal cord. As described previously, the number of PH3+ neural progenitors at E10.5 was not altered by Sema3B depletion. Accordingly, 1-h incorporation of 5-bromodeoxyuridine (BrdU) in the S phase at E11.5 did not reveal significant alteration of the number of cycling neural progenitors up to E11.5 in absence of Sema3B ( Supplementary Fig. 9 ). In contrast, we found that the number of mitotic cells of E11.5 Sema3B −/− spinal cords was 80% of the normal situation both in the dorsal and ventral compartments ( Supplementary Fig. 9 ), suggesting an alteration of cell cycle for a subset of progenitors. As a consequence of this reduced division rate at E11.5, we also observed a decrease in the spinal cord size at E12.5 in Sema3B mutants compared with wild-type littermates ( Supplementary Fig. 9 ). Thus, Sema3B invalidation alters the proliferation and morphogenesis of the spinal cord at E11.5–E12.5. We next assessed neurogenesis defaults. We focused on motor neuron generation, well characterized to occur between E9.5 and E11.5. We observed using Islet1/2+ immunostaining at E12.5 that Sema3B loss did not alter the number of motoneurons ( Supplementary Fig. 9 ). We performed birthdating experiments with BrdU pulse at E10.5 and islet1/2+ immunostaining at E12.5. Motoneurons were born earlier in the wild types as the percentage of Brdu+/Islet1/2+ motor neurons was only 10%, and it increased by twofold in the Sema3B mutants ( Supplementary Fig. 9 ). Thus, loss of access to extracellular Sema3B by dorsal and ventral progenitors at E10.5, at the stage where we detected changes of division orientation, alters the course of proliferation and neurogenesis. Neuropilin 1 and 2 promote planar division in neural progenitors During axon guidance, Sema3B exerts its effects through the receptor Neuropilin 2 (Npn2) [14] , [18] , [26] . However, previous studies showed that Sema3B can also bind with similar affinity to Neuropilin 1 (Npn1), a close relative to Npn2, although its contribution is less documented [26] . Npn1 and Npn2 proteins were detected in the spinal ventricular zone at E10.5 ( Fig. 6 a). We thus investigated the contribution of both Neuropilin receptors in the orientation of cell division in the spinal cord at E10,5. For this purpose, we analysed a Npn2 knockout line [27] and Npn1 knock-in line in which the binding of Sema3s is selectively disrupted [28] . Double homozygous Npn1 Sema/Sema ;Npn2 −/− displayed a significant increase in oblique division percentages compared with wild-type embryos, which mimics Sema3B depletion ( Fig. 6 b). Altogether, these results support the conclusion that Sema3B uses the neuropilin receptors to regulate neural progenitor division orientation. 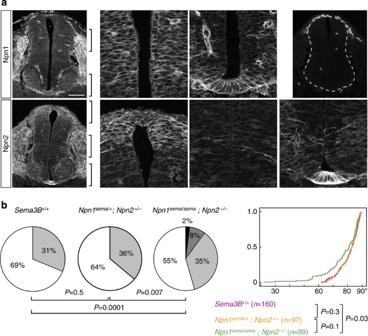Figure 6: Npn1 and Npn2 invalidation alters the orientation of neural progenitor divisions at E10.5. (a) Confocal images showing immunolabelling of Npn1 and Npn2 on spinal cord sections at E10.5. Npn1 and Npn2 proteins are distributed in complementary domains of the VZ. Ctrl-immunostaining without primary antibody. (b) Cumulative fraction curves showing the distribution of neural progenitor division orientation in E10.5Npn1sema/+;Npn2+/−andNpn1sema/sema;Npn2−/−spinal cords (n, number of cells from a minimum of three embryos per conditions from the same litters,Pvalue is from the KS test). The cumulative curve of the E10.5Sema3B+/+condition has been added for comparison. Previous data sets are also displayed in pie charts (Pvalue is from Fisher’s exact test). Figure 6: Npn1 and Npn2 invalidation alters the orientation of neural progenitor divisions at E10.5. ( a ) Confocal images showing immunolabelling of Npn1 and Npn2 on spinal cord sections at E10.5. Npn1 and Npn2 proteins are distributed in complementary domains of the VZ. Ctrl-immunostaining without primary antibody. ( b ) Cumulative fraction curves showing the distribution of neural progenitor division orientation in E10.5 Npn1 sema/+; Npn2 +/− and Npn1 sema/sema; Npn2 −/− spinal cords ( n , number of cells from a minimum of three embryos per conditions from the same litters, P value is from the KS test). The cumulative curve of the E10.5 Sema3B +/+ condition has been added for comparison. Previous data sets are also displayed in pie charts ( P value is from Fisher’s exact test). Full size image Sema3B regulates planar orientation via GSK3 and CRMP2 We next wondered how the function of Sema3B on cell division orientation is achieved. The Semaphorins regulate cell and axon migration through control of cytoskeleton dynamics [29] . Interestingly, altering cortical actin, microtubules and their associated complex NuMA/LGN/Gαi anchoring the mitotic spindle influences the orientation of divisions in the vertebrate spinal cord [16] , [30] . The regulation of cofilin, an actin-depolymerizing protein, through LIMK1-dependent phosphorylation, influences the axon guidance but also mitotic spindle positioning in vitro [31] , [32] . In addition, in Semaphorin-mediated axon guidance, glycogen-synthase Kinase 3β (GSK3β) inactivates through phosphorylation the collapsin response mediator protein 2 (CRMP2), a microtubule-stabilizing protein, thus favouring microtubule depolymerization [33] , [34] , [35] . Several lines of evidence implicate GSK3β in regulating astral microtubule dynamics and spindle orientation [36] , [37] . CRMP members interact with dynein [38] , [39] , a molecular motor also involved in spindle orientation. Previous work showed that inhibiting GSK3 with the selective inhibitor SB216763 alters metaphase progression [40] . We also observed 58% decrease in the proportion of planar divisions in the spinal cord of E10.5 embryos incubated 2 h with SB216763, consistent with a contribution of GSK3 in spindle orientation ( Fig. 7g ). We thus investigated whether Sema3B could act by modulating cofilin and CRMP2 activity in spinal progenitors. We dissected whole spinal cords from wild-type E10.5 embryos, opened them and exposed their surface to Sema3B-Fc. Five-minute treatment decreased the level of cofilin protein, and its form phosphorylated on Ser-3, a target residue of LIMK1 (ref. 41 ; Supplementary Fig. 10 ). In addition, we observed a strong increase in the level of CRMP2 phosphorylated on Thr514 (pCRMP2), a known target of GSK3 (ref. 42 ), after 20-min exposure to Sema3B-Fc compared with control condition ( Fig. 7d and Supplementary Fig. 10 ). To more directly visualize changes of pCRMP2 levels in situ , open books were stimulated with Sema3B-Fc and processed for cryosections and pCRMP2 immunostaining. Predominant pCRMP2 signal was detected in dividing neural progenitors in prophase, metaphase and anaphase ( Fig. 7a,b ). Interestingly, the intensity of pCRMP2 labelling in nonstimulated open books was higher in metaphase cells with planar spindle orientation than those with oblique orientation ( Supplementary Fig. 11 ). We also found that pCRMP2 staining intensity in metaphase increased by 51% after Sema3B treatment ( Fig. 7c,e ). Moreover, this effect was blocked after treatment with SB216763 ( Fig. 7f ). Thus, Sema3B increases the pool of inactive CRMP2 in dividing progenitors in vivo . Finally, to test the contribution of GSK3 in the Sema3B-dependent division plane control, we assayed the angle rescue effects of Sema3B in open-book embryos in presence or absence of the 20-μM GSK3 inhibitor SB216763. Whereas Sema3B exposure restored planar divisions in presence of the DMSO vehicle, the proportion of planar and oblique divisions was not changed by Sema3B in the presence of GSK3 inhibitors ( Fig. 7h ). Consistent results were obtained with 5 μM of SB216763, or with 25 μM of SB415286, another selective GSK3 inhibitor ( Supplementary Fig. 12 ). GSK3 activity is thus required for the Sema3B function in mitotic spindle orientation. 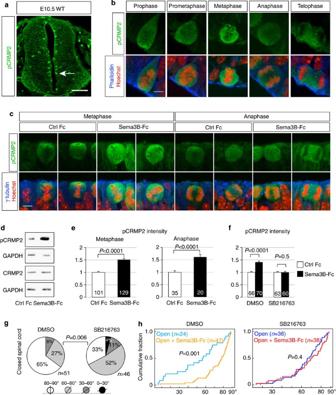Figure 7: Sema3B promotes CRMP2 phosphorylation on Thr514 during metaphase and planar orientation in a GSK3-dependent manner in neural progenitors. (a) Confocal images of anti-phospho-CRMP2 immunostaining of E10.5 spinal cord transverse sections. High level of CRMP2 phosphorylated on Thr514 predominantly accumulates in neural progenitors during mitosis. (b) pCRMP2 was detected in the cytoplasm of mitotic progenitors and strongly accumulated in close vicinity of chromosomes. The pCRMP2 level increases in prophase and metaphase, and then decreases in anaphase and telophase in neural progenitors. (c) Confocal images of anti-phospho-CRMP2, anti-γ-tubulin and Hoechst staining on spinal cord transverse sections of E10.5 embryos in open-book exposed 30 min to Sema3B-Fc or Ctrl Fc. Representative neural progenitors in metaphase and anaphase are shown. (d) Western blot of CRMP2, pCRMP2 and ctrl GAPDH on lysates of E10.5 whole spinal cords exposed 20 min to 5 μg ml−1Sema3B-Fc or Ctrl Fc. (e) Histograms showing the intensity of pCRMP2 staining measured in metaphase and anaphase cells in Sema3B-Fc and Ctrl Fc conditions (n, number of cells from three independent experiments;Pvalue is from Mann–WhitneyU-test). (f) Histograms showing the intensity of pCRMP2 staining measured in metaphase cells of open-book spinal cords treated with Sema3B-Fc and Ctrl Fc following 30′ preincubation with or without the GSK3 inhibitor SB216763. Ind,f, pCRMP2 intensity is expressed relatively to the mean intensity of the respective Ctrl Fc conditions (n, number of cells from three independent experiments;Pvalue is from Mann–WhitneyU-test). (g) Pie charts showing the proportion of planar or oblique divisions of spinal progenitors from E10.5 unopened embryos incubated 2 h with or without 20 μM GSK3 inhibitor SB216763 (n, number of cells from two littermates for each condition;Pis from Fisher’s exact test). (h) Cumulative fraction curves showing the distribution of progenitor division angles in open-book exposed 3 h with or without 5 μg ml−1Sema3B-Fc, in presence of absence of 20 μM GSK3 inhibitor SB216763 (n, number of cells from four embryos for each condition;Pis from the KS test). Sema3B-dependent effects on planar division orientation are blocked by GSK3 inhibitors. Scale bars ina, 100 μm and inb,c, 10 μm. Figure 7: Sema3B promotes CRMP2 phosphorylation on Thr514 during metaphase and planar orientation in a GSK3-dependent manner in neural progenitors. ( a ) Confocal images of anti-phospho-CRMP2 immunostaining of E10.5 spinal cord transverse sections. High level of CRMP2 phosphorylated on Thr514 predominantly accumulates in neural progenitors during mitosis. ( b ) pCRMP2 was detected in the cytoplasm of mitotic progenitors and strongly accumulated in close vicinity of chromosomes. The pCRMP2 level increases in prophase and metaphase, and then decreases in anaphase and telophase in neural progenitors. ( c ) Confocal images of anti-phospho-CRMP2, anti-γ-tubulin and Hoechst staining on spinal cord transverse sections of E10.5 embryos in open-book exposed 30 min to Sema3B-Fc or Ctrl Fc. Representative neural progenitors in metaphase and anaphase are shown. ( d ) Western blot of CRMP2, pCRMP2 and ctrl GAPDH on lysates of E10.5 whole spinal cords exposed 20 min to 5 μg ml −1 Sema3B-Fc or Ctrl Fc. ( e ) Histograms showing the intensity of pCRMP2 staining measured in metaphase and anaphase cells in Sema3B-Fc and Ctrl Fc conditions ( n , number of cells from three independent experiments; P value is from Mann–Whitney U -test). ( f ) Histograms showing the intensity of pCRMP2 staining measured in metaphase cells of open-book spinal cords treated with Sema3B-Fc and Ctrl Fc following 30′ preincubation with or without the GSK3 inhibitor SB216763. In d , f , pCRMP2 intensity is expressed relatively to the mean intensity of the respective Ctrl Fc conditions ( n , number of cells from three independent experiments; P value is from Mann–Whitney U -test). ( g ) Pie charts showing the proportion of planar or oblique divisions of spinal progenitors from E10.5 unopened embryos incubated 2 h with or without 20 μM GSK3 inhibitor SB216763 ( n , number of cells from two littermates for each condition; P is from Fisher’s exact test). ( h ) Cumulative fraction curves showing the distribution of progenitor division angles in open-book exposed 3 h with or without 5 μg ml −1 Sema3B-Fc, in presence of absence of 20 μM GSK3 inhibitor SB216763 ( n , number of cells from four embryos for each condition; P is from the KS test). Sema3B-dependent effects on planar division orientation are blocked by GSK3 inhibitors. Scale bars in a , 100 μm and in b,c , 10 μm. Full size image We then investigated the implication of CRMP2 in mitotic spindle positioning. HeLa cells were transfected with wt, constitutively active (T514A and AAA), phosphomimetic (T514D and DDD) or deleted (ΔC350) mutant forms of CRMP2 (see Methods). Immunostaining of tyrosinated alpha-tubulins [43] was then performed to analyse the organization of astral fibres. Overexpression of wt and mutant CRMP2 forms except ΔC350-CRMP2 strongly disrupted astral microtubules at metaphase. Astral fibres displayed abnormal density and did not properly reach the cell cortex, indicating that manipulating CRMP2 activity affected the astral microtubule turn-over ( Fig. 8a,b ). In addition, overexpression of wt and mutant CRMP2 forms except ΔC350-CRMP2 resulted in delocalization of the mitotic spindle from the cell centre ( Fig. 8c,d ). Finally, we analysed the plane of division of HeLa cells expressing the various CRMP2 forms related to their fibronectin substrate. In the control condition, the vast majority of HeLa cells oriented their metaphase plate orthogonally to the substrate. Whereas the proportion of obliquely dividing HeLa cells already increased after wt and T514D-CRMP2 overexpression compared with controls, the deviation of metaphase plate was even more prominent in the T514A-CRMP2 condition ( Fig. 8e,f ). Thus, manipulation of CRMP2 activity in HeLa cells affects both astral microtubule organization and mitotic spindle orientation. 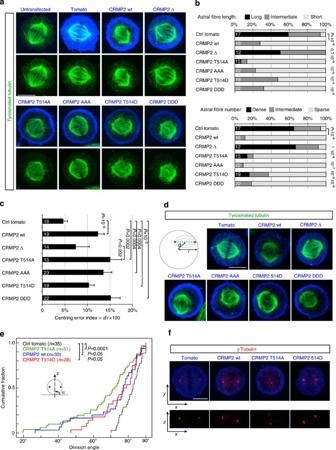Figure 8: CRMP2 has an impact on astral microtubule dynamic, and mitotic spindle positioning. (a) Confocal stack Z projection of tyrosinated Tubulin immunostainings of representative HeLa cells transfected with plasmid expressing ctrl Tomato or CRMP2 mutant forms. Labellings of overexpressed ctrl Tomato or CRMP2 are merged in blue. (b) Histograms showing the percentage of ctrl Tomato or CRMP2 mutant transfected HeLa cells with the indicated astral fibre phenotype. Cells were classified in a blind manner according to two criteria: the number of astral fibres with ‘dense, intermediate and sparse’ classes and the length of astral fibres ‘long’: fibres are long, stretched and anchored to the cortex, ‘intermediate’: fibres are shorter, twisted and do not reach the cell cortex, ‘short’: most fibres are very short or absent (n, number of cells;Pvalue is from Fischer’s exact test; similar results were obtained in two independent experiments). (c) Histograms showing the index of centring error of the mitotic spindle in HeLa transfected with plasmid expressing ctrl Tomato or CRMP2 forms. The centre of the mitotic spindle is the middle of the segment-defined spindle poles. The centring error index is expressed as the percentage of deviation (d) of this point from the cell centre with respect to the cell radius (r) as depicted in the schema (n, number of cells;Pvalue with Mann–WhitneyU-test; similar results were obtained in two independent experiments). (d) Z projection of confocal stacks of tyrosinated Tubulin immunostainings of representative cells in each conditions. Labellings of overexpressed ctrl Tomato or CRMP2 are merged in blue. (e) Cumulative fraction curves showing the distribution of metaphase mitotic spindle angles with respect to the substrate in HeLa cells transfected with plasmid expressing ctrl Tomato or CRMP2 forms and plated on fibronectin-coated coverslips; only cells with identifiable mitotic spindle poles were considered (n, number of cells;Pvalue with the KS test). (f) Z projection (upper) and Y projection (lower) of confocal stacks of γ-Tubulin immunostaining of representative HeLa cells. Labellings of overexpressed ctrl Tomato or CRMP2 are in blue. CRMP2 forms are tagged with myc and revealed with anti-myc immunolabelling (scale bar, 10 μm). Figure 8: CRMP2 has an impact on astral microtubule dynamic, and mitotic spindle positioning. ( a ) Confocal stack Z projection of tyrosinated Tubulin immunostainings of representative HeLa cells transfected with plasmid expressing ctrl Tomato or CRMP2 mutant forms. Labellings of overexpressed ctrl Tomato or CRMP2 are merged in blue. ( b ) Histograms showing the percentage of ctrl Tomato or CRMP2 mutant transfected HeLa cells with the indicated astral fibre phenotype. Cells were classified in a blind manner according to two criteria: the number of astral fibres with ‘dense, intermediate and sparse’ classes and the length of astral fibres ‘long’: fibres are long, stretched and anchored to the cortex, ‘intermediate’: fibres are shorter, twisted and do not reach the cell cortex, ‘short’: most fibres are very short or absent ( n , number of cells; P value is from Fischer’s exact test; similar results were obtained in two independent experiments). ( c ) Histograms showing the index of centring error of the mitotic spindle in HeLa transfected with plasmid expressing ctrl Tomato or CRMP2 forms. The centre of the mitotic spindle is the middle of the segment-defined spindle poles. The centring error index is expressed as the percentage of deviation ( d ) of this point from the cell centre with respect to the cell radius ( r ) as depicted in the schema ( n , number of cells; P value with Mann–Whitney U -test; similar results were obtained in two independent experiments). ( d ) Z projection of confocal stacks of tyrosinated Tubulin immunostainings of representative cells in each conditions. Labellings of overexpressed ctrl Tomato or CRMP2 are merged in blue. ( e ) Cumulative fraction curves showing the distribution of metaphase mitotic spindle angles with respect to the substrate in HeLa cells transfected with plasmid expressing ctrl Tomato or CRMP2 forms and plated on fibronectin-coated coverslips; only cells with identifiable mitotic spindle poles were considered ( n , number of cells; P value with the KS test). ( f ) Z projection (upper) and Y projection (lower) of confocal stacks of γ-Tubulin immunostaining of representative HeLa cells. Labellings of overexpressed ctrl Tomato or CRMP2 are in blue. CRMP2 forms are tagged with myc and revealed with anti-myc immunolabelling (scale bar, 10 μm). Full size image Altogether, this supports that CSF-derived Sema3B likely exerts direct effect on division orientation through a GSK3-CRMP2 pathway having an impact on the dynamic and function of microtubules anchoring the mitotic spindle. In this study, we show that Sema3B, a well-known chemotropic factor, is delivered in the central canal of the neural tube and orients the division of a population of neuroepithelial cells in the vertebrate spinal cord at early steps of neurogenesis ( Fig. 9 ). Our study reveals for the first time that an extracellular signal regulates the orientation of cell division of neural progenitors in the vertebrate nervous system. In other contexts, such extracellular contributions were suspected from studies showing that an asymmetric source of Wnt proteins could orient the division plane of embryonic stem cells in vitro [44] . In epithelial skin tumours, interfering with autocrine loop of vascular endothelial growth factor–Nrp1 in cancer stem cells was also found to alter their division orientation related to the epidermis tissue plane [45] . 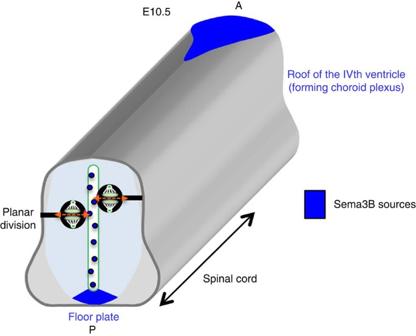Figure 9: Model of Sema3B function proposing that Sema3B is a CSF-derived extracellular signal secreted by the floor plate in the spinal cord and the roof of the IVth ventricle (including the presumptive choroid plexus) in the hindbrain at E10.5. CSF-derived Sema3B promotes the planar orientation of neural progenitor division in the spinal cord. Figure 9: Model of Sema3B function proposing that Sema3B is a CSF-derived extracellular signal secreted by the floor plate in the spinal cord and the roof of the IVth ventricle (including the presumptive choroid plexus) in the hindbrain at E10.5. CSF-derived Sema3B promotes the planar orientation of neural progenitor division in the spinal cord. Full size image Our findings that Sema3B mediates external control of cell division orientation reveal a novel function of chemotropic cues. Such cues were so far essentially known to provide topographic information to migrating cells and axons. We show that they also act at earlier stages during polarized processes of neural progenitors. Our data indicate that Sema3B loss shifts to oblique a fraction of planar divisions. Moreover, short-term exposure of neural progenitors in open-book configuration with Sema3B was sufficient to shift to planar or subplanar a large subsets of oblique divisions. These late and early Semaphorin functions appear to be mediated by a common signalling pathway regulating the microtubule network. We show here that the canonical binding partners of Sema3B, Npn1 and Npn2 are involved in the division orientation of spinal progenitors. Implication of GSK3 and CRMP2, which we found downstream of Sema3B in spinal mitotic progenitors, is also reminiscent of the signalling induced by Semaphorins in differentiating neurons to control their polarity and to collapse their axon growth cones or leading process [33] , [34] , [42] . During the metaphase, the mitotic spindle rotates and is anchored to the lateral cell cortex via dedicated proteins by astral microtubules, and then defining the apicobasal orientation of the division plane [1] , [46] . Interestingly, previous work showed that CRMP2 is specifically associated with spindle and astral microtubules and that CRMP2 knockdown alters astral-microtubule stability [37] , [42] . In this study, we demonstrate that proper CRMP2 activity is required for astral fibre organization and mitotic spindle positioning during metaphase. We also show that endogenous phosphorylated CRMP2 signal is detected in mitotic neural progenitors in metaphase and is strongly increased by apical Sema3B delivery. CSF-derived Sema3B thus likely promotes planar orientation of division via CRMP2-dependent modulation of astral fibre dynamic in neural progenitors. In vivo manipulations of CRMP2 in neural progenitors should be carried out to confirm this model. Various mechanisms can be advanced for future investigations. CSF-derived Sema3B could generate a domain of CRMP2 inactivity and microtubule instability within the apical side of the mitotic progenitor, preventing oblique anchorage of the spindle. Alternatively, Sema3B could restrict the astral microtubule filament length [35] or modulate dynein activity [38] along astral microtubules to constrain the mitotic spindle in the planar position. Loss of Sema3B would then anchor astral microtubules more apically or would introduce laxity of microtubule filaments allowing deviation of the mitotic spindle from the planar orientation. Whether other Semaphorins share this early Sema3B implication is plausible. Expression of other Semaphorins was detected in the spinal cord and in the vicinity of other proliferative zones of the nervous system. In addition, other diffusible guidance cues may influence the orientation of the mitotic spindle. Indeed, several chemotropic factors such as Sonic Hedgehog, Netrin, Slit and Wnt family members are expressed in the floor plate or the roof plate during neurogenesis, some of which being detected in the CSF [47] . Slit members have been shown to promote the proliferation of neural progenitors in the cortex [48] . These secreted factors could contribute to the orientation of progenitor division in a redundant manner. Alternatively, these factors could control specific spatial components of mitotic spindle positioning. Sema3B displays symmetric effect on spindle pole positioning to promote planar orientation. However, since the spindle poles host centrosomes with different ages and composition [49] , extracellular cues could differently affect their positioning. Interestingly, Wnt signalling has been shown to promote spindle size asymmetry leading to unequal division of neural progenitors [50] . Therefore, extracellular cues could set a variety of angles in the various tissue axes through either repulsive or attractive effects. These extracellular factors could also control the orientation of specific subsets of neural progenitors. Previous studies revealed that neural progenitors differing in the division mode and daughter cell fates are intermingled in the spinal neuroepithelium. Such a heterogeneity of progenitors is also reflected in the diversity of their apicobasal division orientations and their responsiveness to Sema3B. Indeed, the shift of planar to oblique divisions consecutive to Sema3B deletion only concerns a part of the progenitor population. Lack of available readouts yet precludes further understanding of the features encoded by such differences of progenitor competence for Sema3B effects and stereotypic distribution of angles. Sema3B might selectively influence a particular type of progenitors within the differently fated populations. Different angle deviations could also correspond to progenitors with different commitment, for example, progenitors, giving rise to one progenitor and one neuron from those giving rise to two progenitors with different fate. Similarly, division orientation could differ between progenitors giving rise to two progenitors fated to undergo division mode similar or different to the mother type. Progenitors giving rise to two neurons and to two progenitors could also divide with slightly different angles [12] . We observed that alteration of the planar/oblique divisions consequent to Sema3B loss is followed by alteration of the spinal cord size and abnormal timing of motoneuron birth. Whether or not the orientation of the progenitor divisions is instructive for cell fate determination in the vertebrate nervous system is still under debate [51] . Besides, a previous characterization of the local spinal cord circuitry revealed that interneurons participating in distinct premotor circuits differ by the timing of their neurogenesis [52] . Functional consequences of the motoneuron birth defects we observed are unknown but could thus have profound impact, which opens fascinating perspectives for future studies. Sema3B and other extracellular cues could therefore play complementary role to that reported for intrinsic polarity in the spindle orientation [1] . Whereas intrinsic polarity cues provide internal landmarks to position the mitotic spindle with respect to the apicobasal axis, extracellular cues such as Sema3B could exert their effect at specific and restricted time window to coordinate the division orientations at the tissue level. This would explain the remarkable stereotypy of the distributions of the division angles that we observed between embryos. Our study allows assigning novel contribution to the floor plate, well known to release morphogens crucial for the dorsoventral patterning of the neuroepithelium [8] . We showed that the floor plate also delivers at the apical pole of the neuroepithelium a Semaphorin signal orienting progenitor divisions along the apicobasal axis. Notably, Sema3B is not restricted to the floor plate but is also synthesized by the choroid plexi in the brain. The CSF is known to convey several patterning and growth-promoting cues for neural progenitor cells in developing and adult brains [53] . Thus, our work opens new lines of investigations and further enlarge the spectrum of neurogenesis processes that could be physiologically and artificially targeted through the CSF. Animals Sema3B −/− mice construct and genotyping have been described previously [14] . Mus musculus Sema3B KO line is in the OF1 background. For the construction of the Sema3B-GFP KI allele, the coding sequence of eGFP (Clontech) was fused to the N-terminal part of Sema3B. The Sema3B-GFP KI was generated in the C57bl/6 background ( Supplementary Fig. 4 ). Sema3B-GFP mice were genotyped with the following set of primers: Sema3Ba, Sema3Bb (ref. 14 ) and GFP-AS (CGCCGATGGGGGTGTTCTGC). The PGK:Cre; Dbx1-IRES-loxP-Stop-loxP-DTA mouse line has been described previously [20] . Neuropilin1 Sema/Sema and Neuropilin2 −/− mouse construct and genotyping have been described previously [27] , [28] . Animals were handled according to the french national regulations, and the protocols were validated by the European Research Council ethical committee In situ hybridization In situ hybridization was carried out on 20-μm cryosections from gelatine/sucrose-embedded embryos, as described previously [54] . Immunofluorescent labelling Whole-mounted embryo and 30-μm cryostat sections were incubated for 3 h or 1 h, respectively, in a blocking solution (2% BSA and 0.5%Triton X-100 in PBS) and incubated with primary antibodies diluted in the blocking solution. The primary antibodies used were a rat anti-phospho-Histone PH3 (ref. 55 ; HTA28; Sigma Aldrich; 1:50), mouse anti-γ-tubulin [56] (GTU-88; Sigma Aldrich; 1:100) and anti-acetylated tubulin (Sigma Aldrich; 1:100), rat anti-tyrosinated Tubulin [57] (YL1/2, Santa Cruz Biotechnology; 1:200), rabbit anti-GFP (A6455; Invitrogen; 1:100), rabbit anti-ZO1 (ref. 58 ; Zymed Laboratories; 1:100), rabbit anti-aPKC (sc-216, Santa Cruz Biotechnology; 1:100), rabbit anti-Olig2 (ref. 59 ; AB9610 Chemicon, Millipore; 1:100), rabbit anti-phosphoThr514-CRMP2 (refs 60 , 61 ; ab62478; Abcam; 1:100), rabbit anti-CRMP2 (9393, Cell Signaling Technology; 1:1,000), mouse anti-cMyc (9E10, Sigma Aldrich; 1:100), and goat anti-Npn1 and anti-Npn2 (AF566 and AF567 R&D, 1/50). Mouse monoclonal anti-Nkx2.2 (74.5A5; 1:50), anti-Nkx6.1(F55A10; 1:50) and anti-Pax7 (1:50) were from the Developmental Studies Hybridoma Bank. Embryos and sections were then incubated with suitable fluorescent secondary antibodies. Secondary antibodies were Texas-red anti-rat (Jackson Immuno-research), Alexa488 anti-rat, anti-mouse and anti-rabbit, Alexa555 anti-rabbit, Alexa647 anti-rabbit and anti-mouse (Molecular Probes) and Fluoprobes547 anti-mouse (Interchim). Cell nuclei were stained with bisbenzimide (Promega) and F-actin was stained with TRITC-phalloidin (Sigma Aldrich). Staining was observed under Zeiss LSM510 or Olympus FV1000 confocal microscopes. ‘Open-book’ surgery The neural tube of OF1 mouse embryos was dorsally incised in «Open-Book» configuration with fine needles. It is then freely opened without stretching. The apical surface of the neuroepithelium was thoroughly rinsed and were subsequently incubated for 3 h in a specific medium composed of 1:1 DMEM/F12-Neurobasal medium supplemented with N2, B27 supplements diluted to 0.5x (Gibco). For rescue experiments, carrier-free Sema3B-Fc chimera protein (R&D Systems) was added to the above medium. For anti-phospho-CRMP2 immunostaining, open-book embryos were pre-incubated 30 min in presence or absence of 5–25 μM selective GSK3 inhibitors SB216763 and SB415286 (Tocris), and then incubated for 30 min with 5 μg ml −1 Fc or Sema3B-Fc in DMEM-Glutamax with (Gibco). For division orientation analysis, open-book embryos were incubated for 2 h 30 min with Sema3B-Fc or Ctrl following GSK3 inhibitor treatment. Quantifications For cell division angle measurement, as the mitotic spindle undergoes rapid rotations during metaphase and is stabilized at anaphase [62] , PH3+ anaphase cells were analysed. High-magnification 3D stacks of anaphase cells were obtained from transverse sections using confocal microscopy. The acquisitions were performed at the brachial, thoracic and lumbar levels of the spinal cord, in similar manner under each condition. The angle analysis was performed in a blind manner. The cartesian ( x , y , z ) coordinates of both centrosomes (γ-tubulin+; C and C′) and three points delineating the apical plane (A1, A2 and A3) were measured with the ImageJ software. The three points of the apical plane were used to calculate the coordinates of the vector orthogonal (normal) to this plane. The normal vector to the division plane was deduced from the coordinates of the two centrosomes. The angle ( α) between the apical plane and the division plane was calculated using the following formula: COS( α )=|( x C′ − x C )(( y A2 − y A1 )( z A3 − z A1 )−( y A3 − y A1 )( z A2 − z A1 ))+( y C′ − y C )(( x A3 − x A1 )( z A2 − z A1 )−( x A2 − x A1 )( z A3 − z A1 ))+( z C′ − z C )(( x A2 − x A1 )( y A3 − y A1 )−( x A3 − x A1 )( y A2 − y A1 ))/( ✓ (( y A2 − y A1 ) × ( z A3 − z A1 )−( y A3 − y A1 ) × ( z A2 − z A1 )) 2 +(( x A3 − x A1 ) × ( z A2 − z A1 )−( x A2 − x A1 ) × ( z A3 − z A1 )) 2 +(( x A2 − x A1 ) × ( y A3 − y A1 )−( x A3 − x A1 ) × ( y A2 − y A1 )) 2 × ✓ (( x C′ − x C ) 2 +( y C′ − y C ) 2 +( z C′ − z C ) 2 )|. The number of PH3+ cells normalized by spinal cord height gives the mitotic index. The proportion of cells in pro/meta/anaphase was expressed as a percentage of the PH3+ cells. HeLa cell culture and transfection HeLa cells (ATCC) were cultured in DMEM with 10% fetal calf serum (FCS; Invitrogen). HeLa cells were grown on glass coverslips and transfected 4 h with the Jet prime Kit (Polyplus) according to the manufacturer’s instructions, and were fixed 24 h later in 4% paraformaldehyde (PFA). Plasmids expressing wild-type and mutant forms of myc-tagged human CRMP2 were described previously. In the T514D and T514A-CRMP2 forms, the GSK3-phosphorylated Threonine 514 was replaced by phosphomimetic and non-phosphorylable residues, respectively. The three phosphorylation sites T514, S518 and S522 were mutated in AAA and DDD-CRMP2 (ref. 42 ). In the ΔC350-CRMP2 form (here referred as ΔCRMP2), domains interacting with microtubules, kinesins and Sra-1 are lost [38] . For immunofluorescent labelling, antibodies were diluted in 3% BSA, 0.5% Tween20 and PBS. Conditioned media For Sema3B cm and ctrl cm , HEK293T cells (ATCC; certified by the company) were transfected with plasmids encoding either Sema3B-GFP fusion protein, Sema3B-Alkaline Phosphatase fusion, control GFP or AP proteins. The conditioned medium was produced in DMEM-Glutamax with 10% FCS (Invitrogen). For FP cm , floor plates (FPs) were isolated from OF1 and Sema3B-GFP KI E12.5 embryos and were cultivated in 0.5% low melting agarose (Sigma Aldrich) clots in B27-supplemented Neurobasal medium. Dot blot and western blot analyses FP cm from E12.5 WT and Sema3B gfp embryos were spotted on a nitrocellulose membrane and were probed with mouse anti-GFP antibody (A6455; Invitrogen; 1/1,000). CSF was harvested in the IVth ventricle of mouse E10.5 embryos with pulled glass micropipettes. The CSF was then processed for western blot analysis using anti-GFP antibody (1/1,000). Whole spinal cords were carefully dissected from E10.5 wild-type embryos at 4 °C, randomly allocated into two groups and then incubated for 5 or 20 min with Sema3B-Fc or ctrl IgG-Fc (5 μg ml −1 ; R&D) in DMEM-Glutamax (Invitrogen) at 37 °C. Spinal cords were then rinsed at 4 °C and lysed in lysis buffer containing Phostop phosphatase inhibitors (Roche). Protein lysates were analysed using western blot with a rabbit anti-phospho-Cofilin antibody targeted against the phosphorylated Ser-3 (no. 3311 Cell Signaling Technology, 1/1,000), a rabbit anti-Cofilin (total) antibody (no. 3312 Cell Signaling Technology, 1/1,000), a rabbit anti-phospho-CRMP2 antibody directed against the phosphorylated Thr514 (ref. 63 ; Abcam, 1/1,000) and a rabbit anti-CRMP2 (total) antibody [63] (no. 9393 Cell Signaling Technology, 1/1,000). Anti-GAPDH antibody (Cell Signaling Technology) was used for loading control. Suitable peroxydase-coupled secondary antibodies (Jackson Laboratories) diluted in PBS-5% BSA were used. Membranes were revealed with chemiluminescence with Clarity western ECL (Bio-Rad). Chemiluminescence was acquired with Chemidoc (Bio-Rad). Ratio between Cofilin or CRMP2 staining and internal GAPDH staining was assessed with ImageLab (Bio-Rad). Binding experiments Sema3B-GFP and Ctrl GFP conditioned media were concentrated 60 times on amicon columns (Millipore), and their final concentration was assessed with anti-GFP dot blotting. A clusterization step was performed by incubation of the conditioned medium with 10 μg ml −1 rabbit anti-GFP antibodies (Invitrogen) for 1 h at 37 °C. Binding was performed either on cryostat sections of frozen E10.5 embryos or on whole mount embryos freshly dissected in open-book configuration in DMEM-Glutamax. Fresh cryosections were incubated for 1 h at room temperature and open books for 30 min at 10 °C in blocking solution (10% FCS in PBS with 4 mM MgCl 2 and 4 mM CaCl 2 ). Cryosections and open books were then incubated with clustered probes for 1 h and 30 min, respectively, at room temperature or 37 °C, then rinsed and fixed in 4% PFA. Immunostaining of anti-GFP antibodies was then performed with suitable Alexa488 secondary antibodies as described previously. Statistical analysis Statistics analyses were performed with the R software. The nonparametric Mann–Whitney U -test (two-tailed) was used for mitotic index, area and intensity analyses. Fisher’s exact test and Kolmogorov–Smirnov test (two-tailed) were used for comparison of angle value distributions. Fisher’s exact test (two-tailed) was used for comparison of mitotic phase distributions. Error bars correspond to s.e.m. P values are indicated on graphs. Samples were processed in a random manner in in vivo , ex vivo or in vitro experiments. No samples were excluded before statistical analyses. How to cite this article: Arbeille, E. et al. Cerebrospinal fluid-derived Semaphorin3B orients neuroepithelial cell divisions in the apicobasal axis. Nat. Commun. 6:6366 doi: 10.1038/ncomms7366 (2015).